Forced protein unfolding leads to highly elastic and tough protein hydrogels Protein-based hydrogels usually do not exhibit high stretchability or toughness, significantly limiting the scope of their potential biomedical applications. Here we report the engineering of a chemically cross-linked, highly elastic and tough protein hydrogel using a mechanically extremely labile, de novo -designed protein that assumes the classical ferredoxin-like fold structure. Due to the low mechanical stability of the ferredoxin-like fold structure, swelling of hydrogels causes a significant fraction of the folded domains to unfold. Subsequent collapse and aggregation of unfolded ferredoxin-like domains leads to intertwining of physically and chemically cross-linked networks, entailing hydrogels with unusual physical and mechanical properties: a negative swelling ratio, high stretchability and toughness. These hydrogels can withstand an average strain of 450% before breaking and show massive energy dissipation. Upon relaxation, refolding of the ferredoxin-like domains enables the hydrogel to recover its massive hysteresis. This novel biomaterial may expand the scope of hydrogel applications in tissue engineering. Due to their potential applications in biomedical and tissue engineering, protein-based hydrogels have attracted considerable interest [1] , [2] . Most synthetic proteinaceous hydrogels are constructed from unstructured or non-globular proteins [3] , [4] , [5] , [6] , [7] , [8] , [9] , [10] and usually do not exhibit high stretchability or toughness, significantly limiting the scope of their applications. However, folded globular proteins are found in a wide range of naturally occurring biological materials. Force-induced unfolding of proteins can lead to a large extension of the polypeptide chain and result in effective energy dissipation [11] , [12] , [13] , [14] , [15] . Many biological systems, such as fibrin clots [16] , muscles [11] , [17] , [18] and extracellular matrices [14] , [19] have effectively exploited such features to achieve desirable mechanical properties and regulate their biological functions. For example, unfolding a small number of folded domains in the giant muscle protein titin effectively dissipates energy and prevents damage to the tissues by overstretching [17] , [18] . The forced unfolding of fibrinogen has been proposed to be responsible for the marked extensibility, water loss and negative compressibility of fibrin gels [16] . As such, forced protein unfolding offers an attractive strategy to design protein hydrogels that are highly stretchable and tough if a significant degree of protein unfolding can be triggered in hydrogels on the macroscopic scale. However, it is extremely challenging to trigger the forced unfolding of a significant fraction of proteins in hydrogels on the macroscopic scale, and thus such unique features have not been explored in the design of protein-based biomaterials with exceptional mechanical properties. One of the challenges in engineering such materials is that the force experienced by individual polymer chains that compose hydrogels is small; theoretical estimations suggest that the force experienced by individual molecules is on the order of a few picoNewtons (pN) even at intermediate hydrogel deformation (with a strain of 100–200%) [20] . In contrast, forced unfolding of typical elastomeric proteins may require tens or even hundreds of pN [21] . Thus, forced unfolding will only occur for a very small number of proteins in hydrogels constructed using such elastomeric proteins, such as the protein hydrogels we constructed to mimic the passive elastic properties of muscles [22] . Here, to overcome these challenges, we propose to use extremely mechanically labile proteins as building blocks in order to trigger large-scale protein unfolding in hydrogels. Using this design principle, we report the engineering of a highly elastic and tough protein hydrogel based on a de novo -designed protein that assumes the classical ferredoxin-like fold structure (FL). We show that FL-based artificial elastomeric proteins can be photochemically cross-linked and cast into solid hydrogels. The swelling of the hydrogel results in force-induced unfolding of a large fraction of FL domains, which is confirmed by cysteine shotgun fluorescence labelling and mass spectrometry. Subsequent collapse and aggregation of unfolded FL domains leads to intertwining of physically and chemically cross-linked networks, entailing hydrogels with unusual physical and mechanical properties: a negative swelling ratio and opaque appearance, high stretchability and toughness. Our study demonstrates the feasibility of molecular level engineering of protein hydrogels with exceptional properties that may expand the scope of hydrogel applications in tissue engineering. The designed FL domain is mechanically labile In order to find promising candidate proteins that are extremely mechanically labile and can serve as building blocks to engineer protein-based biomaterials, we surveyed the mechanical stability of proteins in the literature as well as proteins that we use to study mechanical unfolding pathways in our laboratories via single-molecule atomic force microscopy (AFM) [11] , [23] and optical tweezers [24] , [25] . The size of these proteins ranges from 50 residues to close to 300 residues, and the majority of them are around 90 residues long [21] , [26] . Through these efforts, we found that a de novo -designed protein, termed as the FL domain (owing to its ferredoxin-like fold structure), exhibits lowest mechanical stability among the proteins we have surveyed and is a promising candidate. FL consists of 82 residues and is a computationally redesigned variant of a previously reported successful designer protein Di-I_5 (PDB code: 2KL8) [27] . FL and Di-I_5 share high sequence identity (75%). Computational modelling predicted that FL folds into a three-dimensional structure that is highly homologous to that of Di-I_5. As shown in Fig. 1a , the predicted structure of FL assumes the classic ferredoxin-like fold with the signature βαββαβ secondary structure arrangement along its backbone. Compared with DI-I_5, FL is thermodynamically less stable (with a of 3.8 kCal mol −1 versus 9.1 kCal mol −1 for DI-I_5) [27] . 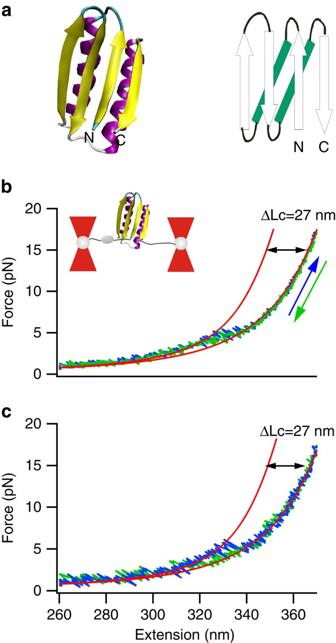Figure 1: Optical trapping experiments reveal that FL is mechanically labile. (a) The predicted three-dimensional structure of the FL domain (left) and its schematic representation (right). The FL domain assumes the classic ferredoxin-like fold with the signature βαββαβ secondary structure arrangement along its backbone. In the schematic, open arrows represent β strands, green boxes represent α-helices and black lines indicate loops between secondary structure elements. (b,c). Representative force–extension curves of a single-FL domain (b: pulling velocity of 100 nm s−1;c: pulling velocity of 500 nm s−1). The distinct unfolding force peak, occurring at∼5 pN with a contour length incrementΔLc of∼27 nm, corresponds to the unfolding of a FL domain. Red lines correspond to fits to the experimental data using the extendable worm-like chain model of polymer elasticity. The relaxation curves show that FL can refold when the stretching force is relaxed. Inset: schematic of the optical trapping geometry with the FL domain linked via DNA handles to functionalized silica beads. The predicted three-dimensional structure of the FL domain shows an α/β structure that belongs to the ferredoxin-like fold. As the N, C-termini of FL is close to each other, we added a mechanically stable GB1 domain (grey ellipsoid) at the N terminus of FL to facilitate the attachment of DNA handles to FLviacysteine cross-linking. The schematic is not drawn to scale. Figure 1b,c shows representative force–extension relationships of FL flanked by two long DNA duplex handles measured on a dual-trap optical tweezers setup [25] . Evidently, the mechanical unfolding of FL occurs at ∼ 5 pN and exhibits a contour length increment (ΔLc) of ∼ 27 nm, which is in good agreement with the expected ΔLc of FL. Calculations based on constant–distance measurements show that the ΔG U–F at zero force is 3.6±0.4 kCal mol −1 for the forced mechanical unfolding of FL (see Supplementary Fig. S1 ), which is close to the measured from chemical unfolding experiments. This result indicates that FL is extremely mechanically labile and only 5 pN of force is sufficient to unfold FL, making FL an ideal candidate for engineering protein hydrogels with unusual mechanical properties. Figure 1: Optical trapping experiments reveal that FL is mechanically labile. ( a ) The predicted three-dimensional structure of the FL domain (left) and its schematic representation (right). The FL domain assumes the classic ferredoxin-like fold with the signature βαββαβ secondary structure arrangement along its backbone. In the schematic, open arrows represent β strands, green boxes represent α-helices and black lines indicate loops between secondary structure elements. ( b , c ). Representative force–extension curves of a single-FL domain ( b : pulling velocity of 100 nm s −1 ; c : pulling velocity of 500 nm s −1 ). The distinct unfolding force peak, occurring at ∼ 5 pN with a contour length increment Δ Lc of ∼ 27 nm, corresponds to the unfolding of a FL domain. Red lines correspond to fits to the experimental data using the extendable worm-like chain model of polymer elasticity. The relaxation curves show that FL can refold when the stretching force is relaxed. Inset: schematic of the optical trapping geometry with the FL domain linked via DNA handles to functionalized silica beads. The predicted three-dimensional structure of the FL domain shows an α/β structure that belongs to the ferredoxin-like fold. As the N, C-termini of FL is close to each other, we added a mechanically stable GB1 domain (grey ellipsoid) at the N terminus of FL to facilitate the attachment of DNA handles to FL via cysteine cross-linking. The schematic is not drawn to scale. Full size image The extremely low mechanical stability of FL is consistent with its structural topology. In the three-dimensional structure of FL, two terminal force-bearing β-strands are next to each other and arranged in an antiparallel fashion. Upon stretching, the two β-strands will be stretched in an unzipping fashion, constituting a typical unzipping topology in which backbone hydrogen bonds connecting the two force-bearing β-strands will be ruptured sequentially. These features are typical of mechanically labile proteins [21] , [26] , [28] . However, it is important to note that these topological features can only give qualitative estimations of the mechanical stability of proteins, and quantitative prediction remains challenging. (FL) 8 -based hydrogels are opaque and show negative swelling Using well-established protein engineering techniques [13] , we engineered a tandem modular protein (FL) 8 , containing eight FL domains arranged in tandem. The polyprotein can be expressed and purified with high yield ( ∼ 80 mg l −1 of bacterial culture) (see Supplementary Fig. S2 ). To engineer (FL) 8 -based hydrogels, we employed the well-developed [Ru(bpy) 3 ] 2+ -mediated photochemical cross-linking strategy [4] , [22] , [29] , which allows the cross-linking of two tyrosine residues in close proximity into a dityrosine adduct and has previously been used to successfully cross-link a range of proteins into protein hydrogels [4] , [22] , [30] , [31] , [33] , [34] , [35] . Each FL domain contains two exposed tyrosine residues, allowing for the possibility of cross-linking utilizing this strategy. We found that upon illumination under white light, concentrated (FL) 8 polyprotein solution in phosphate-buffered saline (PBS) (>100 mg ml −1 ) can be readily cross-linked into solid hydrogels with an opaque appearance at room temperature. 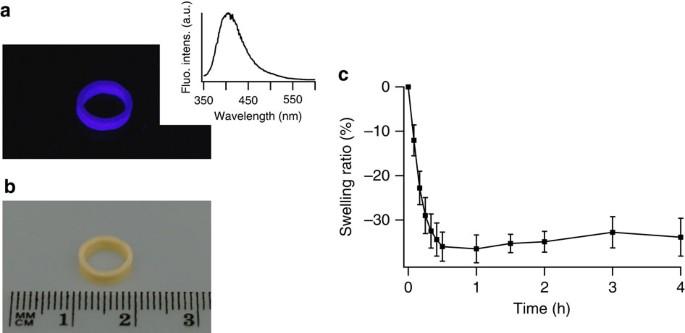Figure 2: Hydrogels made of the (FL)8polyprotein show unusual physical properties. (a) Photographs of moulded rings constructed from (FL)8under ultraviolet illumination. The inset is the fluorescence spectrum of the (FL)8hydrogel. The blue fluorescence under ultraviolet illumination originates from dityrosine cross-links in the hydrogels. (b) Photographs of moulded rings constructed from (FL)8under white light. illumination. (FL)8-based hydrogels are opaque. (c) (FL)8-based hydrogels show spontaneous water expulsion. When soaked in PBS, (FL)8-based hydrogels spontaneously lose water, resulting in a negative swelling ratio of the hydrogel. Error bars represent s.d. of the experimental data. Figure 2a,b shows optical photographs of moulded rings of (FL) 8 . The formation of dityrosine cross-links is evidenced by their strong characteristic blue fluorescence (with an emission wavelength of ∼ 410 nm) upon ultraviolet irradiation [4] , [22] ( Fig. 2a , inset). The opaque appearance of (FL) 8 hydrogels suggests the formation of large aggregated structures in the FL hydrogels, which can scatter light and give rise to an opaque appearance. Figure 2: Hydrogels made of the (FL) 8 polyprotein show unusual physical properties. ( a ) Photographs of moulded rings constructed from (FL) 8 under ultraviolet illumination. The inset is the fluorescence spectrum of the (FL) 8 hydrogel. The blue fluorescence under ultraviolet illumination originates from dityrosine cross-links in the hydrogels. ( b ) Photographs of moulded rings constructed from (FL) 8 under white light. illumination. (FL) 8 -based hydrogels are opaque. ( c ) (FL) 8 -based hydrogels show spontaneous water expulsion. When soaked in PBS, (FL) 8 -based hydrogels spontaneously lose water, resulting in a negative swelling ratio of the hydrogel. Error bars represent s.d. of the experimental data. Full size image In addition to its opaque appearance, FL-based hydrogels also exhibit a surprising ‘deswelling’ behaviour in PBS buffer. When soaked in PBS, most protein hydrogels swell due to favourable interactions between constituent proteins and water, as water is a good solvent for folded proteins. In contrast, FL hydrogels ‘deswell’ in PBS, resulting in a ∼ 34% decrease in volume. Additionally, the FL hydrogel loses ∼ 35% of its original weight by spontaneous water expulsion during this process ( Fig. 2c ). Such deswelling behaviors observed here for the (FL) 8 hydrogel in PBS are unusual for protein-based hydrogels. It is of note that the deswelling process is slow and occurs on a time scale of 10 minutes. These unique properties, which are indicative of conformational changes of FL occurring in hydrogels, are somewhat reminiscent of those arising from the collapse of polymer gels [36] , [37] and hydrophobic collapse and aggregation of unfolded polypeptides. Water loss during stretching has been observed in fibrin clots [16] , for which forced unfolding of fibrinogen has been suggested to be responsible. Considering the force generated during the swelling of protein hydrogels and the extremely low mechanical stability of FL domains, we speculate that forced unfolding of FL domains in the hydrogel may be the origin of these unique macroscopic properties. To investigate the microstructure of these hydrogels, we carried out scanning electron microscopy (SEM) experiments. The hydrogel shows an interconnected porous network structure, as observed using SEM after the hydrogel was shock-frozen ( Fig. 3 ). Compared with hydrogels before deswelling ( Fig. 3a ), deswelled hydrogels appear to have shrunk, and show more rugged and aggregated structures ( Fig. 3b ). This observation is consistent with the deswelling of hydrogels. However, it is not possible to pinpoint the microaggregates formed by the force-induced unfolded FL domains. Direct observation of such microaggregates would require methods that can unambiguously distinguish folded and unfolded proteins in the hydrogels. 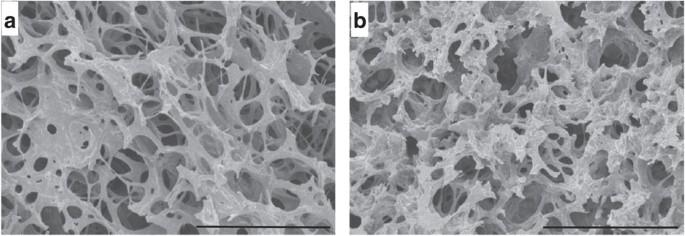Figure 3: SEM images of (FL)8-based hydrogels. (a) before deswelling; (b) after deswelling. The SEM experiments showed that FL hydrogels show typical interconnected, porous structures with the pore size on the scale of a few micrometres. Compared with hydrogels before deswelling (a), deswelled hydrogels (b) appear to have shrunk, and show more rugged and aggregated structures. This observation is consistent with the deswelling of hydrogels. Figure 3: SEM images of (FL) 8 -based hydrogels. ( a ) before deswelling; ( b ) after deswelling. The SEM experiments showed that FL hydrogels show typical interconnected, porous structures with the pore size on the scale of a few micrometres. Compared with hydrogels before deswelling ( a ), deswelled hydrogels ( b ) appear to have shrunk, and show more rugged and aggregated structures. This observation is consistent with the deswelling of hydrogels. Full size image A large fraction of FL domains in hydrogels is unfolded To directly investigate whether some FL domains are indeed unfolded in the hydrogels, we employed the Cysteine shotgun approach to label sterically shielded cysteines with fluorescent dyes in situ [38] . This method has been used to directly demonstrate forced unfolding of proteins in a range of systems under stress, such as red blood cells [38] , [39] and extracellular matrix proteins [19] . FL does not contain endogeneous cysteine residues. Therefore, we mutated a buried Met23 residue to Cys in FL. This mutation does not change the secondary structure of FL and only slightly affects its thermodynamic stability (see Supplementary Fig. S3 ). Hydrogels made of (FL-M23C) 8 showed similar physical properties as those made of wild-type FL (see Supplementary Fig. S4 ). In the folded state, Cys23 is buried in the hydrophobic core and not accessible for fluorophore labelling in solution ( Fig. 4a,b ). However, upon unfolding, Cys23 becomes exposed and can be labelled by thioreactive dyes. We used the small fluorescent dye IAEDANS (5-((((2-iodoacetyl)amino)ethyl)amino) naphthalene-1-sulphonic acid) for Cysteine shotgun labelling, which gives characteristic greenish blue fluorescence at 490 nm when excited at 336 nm ( Fig. 4a ). We utilized this method to test whether certain fraction of FL-M23C are indeed unfolded in the hydrogel ( Fig. 4c,d ). As expected, the FL-M23C hydrogels in PBS buffer shows strong greenish blue fluorescence after shot labelling using IAEDANS. Fluorescence emission spectrum of the FL-M23C hydrogels confirms that the greenish blue fluorescence indeed originates from IAEDANS, indicating that some FL-M23C domains are indeed unfolded in the hydrogel, making some of the cysteine residues accessible for fluorescent dye labelling. Experiments using liquid chromatography-coupled tandem fourier transform mass spectrometer allowed us to identify the labelled peptide from trypsin digested FL-M23C hydrogels (see Supplementary Fig. S5 ), further confirming that some FL-M23C domains are indeed unfolded in the hydrogel. Using the fluorescence intensity of IAEDANS-labelled and completely denatured FL-Met23C hydrogels as a reference, we estimated that ∼ 30% FL-Met23C domains are unfolded in the hydrogels after swelling ( Fig. 4e ). These results strongly indicate that the unfolding of a significant fraction of FL domains and possibly their subsequent collapse/aggregation in the hydrogel are likely responsible for unusual physical properties of FL hydrogels. However, it is important to note that direct evidence at the molecular level for the aggregation of unfolded FL domains is still needed, although the opaque appearance of FL hydrogels provides clear indication of the formation of large aggregates. In principle, repeated unfolding–refolding experiments of (FL) 8 using single-molecule force spectroscopy should be able to provide direct evidence for the aggregation. However, deswelling experiments indicated that the aggregation is a slow process (with a rate constant of 0.09 min −1 , assuming first-order kinetics, Fig. 2c ). Such slow kinetics are very difficult to monitor using the current force spectroscopy instrumentation, due to limited long-term stability. Indeed, in our repeated unfolding–refolding experiments on (FL) 8 using AFM, we did not observe aggregation within the longest relaxation time (1 min) in our AFM, consistent with the slow kinetics suggested by deswelling experiments. 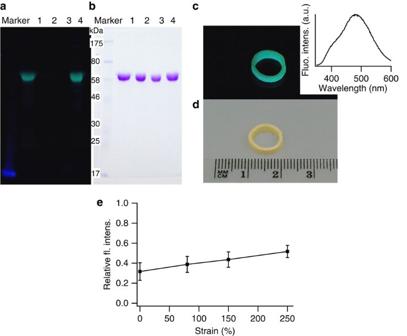Figure 4: Cysteine shotgun labelling experiments. (a,b). SDS–PAGE shows that Cys23 is buried in the folded state and becomes exposed only after FL-M23C is denatured.ais under ultraviolet illumination andbis under white light. Lane 1: molecular weight marker; lane 2: (FL-M23C)8, denatured in 7M GuHCl and labelled by IAEDANS; lane 3: (FL-M23C)8, reacted with IAEDANS in its native conformation; lane 4: (FL)8, reacted with IAEDANS (negative control); lane 5: (FL-C)8, reacted with IAEDANS in the native state (positive control). FL-C contains a C-terminal cysteine residue as well as a N-terminal cysteine residue, which are always exposed. (c) Photographs of (FL-M23C)8hydrogels labelled with IAEDANS in PBS buffer under ultraviolet illumination. The inset is the fluorescence spectrum of the (FL-M23C)8hydrogel labelled with IAEDANS. The dominant peak at 490 nm is characteristic of IAEDANS, while the shoulder peak at 410 nm originates from the dityrosine fluorescence. The characteristic greenish blue fluorescence of (FL-M23C)8hydrogels strongly indicates that some FL-M23C domains are unfolded in the hydrogel. (d) Photographs of (FL-M23C)8hydrogels labelled with IAEDANS in PBS buffer under white light. (e) Estimate of fraction of FL domains that are unfolded in the hydrogels by using the relative fluorescence intensity of IAEDANS-labelled hydrogels. In this measurement, the IAEDANS fluorescence intensity at 490 nm of dye-labelled, completely denatured FL-M23C hydrogels was taken as one, and the fluorescence intensity at 490 nm of unlabelled hydrogels was taken as zero. Assuming that the fluorescence intensity is linearly proportional to the concentration of IAEDANS-labelled FL, we calculated that∼30% of FL domains are unfolded in the unstrained hydrogels. In addition, the fraction of unfolded FL domains increases as a function of strain. Error bars represent s.d. of the experimental data. Figure 4: Cysteine shotgun labelling experiments. ( a , b ). SDS–PAGE shows that Cys23 is buried in the folded state and becomes exposed only after FL-M23C is denatured. a is under ultraviolet illumination and b is under white light. Lane 1: molecular weight marker; lane 2: (FL-M23C) 8 , denatured in 7M GuHCl and labelled by IAEDANS; lane 3: (FL-M23C) 8 , reacted with IAEDANS in its native conformation; lane 4: (FL) 8 , reacted with IAEDANS (negative control); lane 5: (FL-C) 8 , reacted with IAEDANS in the native state (positive control). FL-C contains a C-terminal cysteine residue as well as a N-terminal cysteine residue, which are always exposed. ( c ) Photographs of (FL-M23C) 8 hydrogels labelled with IAEDANS in PBS buffer under ultraviolet illumination. The inset is the fluorescence spectrum of the (FL-M23C) 8 hydrogel labelled with IAEDANS. The dominant peak at 490 nm is characteristic of IAEDANS, while the shoulder peak at 410 nm originates from the dityrosine fluorescence. The characteristic greenish blue fluorescence of (FL-M23C) 8 hydrogels strongly indicates that some FL-M23C domains are unfolded in the hydrogel. ( d ) Photographs of (FL-M23C) 8 hydrogels labelled with IAEDANS in PBS buffer under white light. ( e ) Estimate of fraction of FL domains that are unfolded in the hydrogels by using the relative fluorescence intensity of IAEDANS-labelled hydrogels. In this measurement, the IAEDANS fluorescence intensity at 490 nm of dye-labelled, completely denatured FL-M23C hydrogels was taken as one, and the fluorescence intensity at 490 nm of unlabelled hydrogels was taken as zero. Assuming that the fluorescence intensity is linearly proportional to the concentration of IAEDANS-labelled FL, we calculated that ∼ 30% of FL domains are unfolded in the unstrained hydrogels. In addition, the fraction of unfolded FL domains increases as a function of strain. Error bars represent s.d. of the experimental data. Full size image (FL) 8 -based hydrogels show excellent mechanical properties Having confirmed that a significant fraction of FL domains are already unfolded and aggregated in the hydrogel, we then carried out tensile measurements to test the mechanical properties of these hydrogels in PBS at room temperature. For technical considerations, we used ring-shaped samples for tensile testing [40] . Typical stress-strain curves of (FL) 8 -based hydrogels are shown in Fig. 5 . We found that although this hydrogel contains 70% water, it is highly elastic and can be stretched to >5 times its original length without breaking ( Fig. 5a ), giving rise to an average breaking strain of 450±90 ( n =16, data are represented as average±standard deviation (s.d.)) with a Young’s modulus at 15% strain of 16±3 kPa ( n =27, measured on the very first stress-strain curves). In addition, these hydrogels show remarkable hysteresis between stretching and relaxation cycles ( Figs. 5b,c ), suggestive of large energy dissipation. When FL hydrogels are subject to consecutive stretching–relaxation cycles with increasing strains, they show significant quasi-plastic deformation when stretched to higher strains ( Fig. 5b ). The FL hydrogels demonstrate a fracture stress of 35±6 kPa ( n =16). It is of note that hydrogels constructed from FL-M23C exhibit similar mechanical properties (see Supplementary Fig. S6 ). 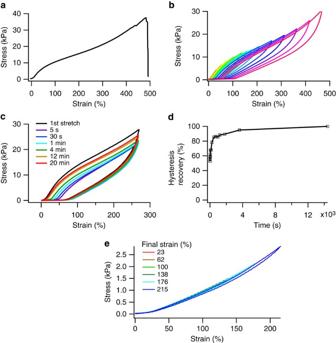Figure 5: Mechanical properties of (FL)8hydrogels. (a) Representative stress-strain curve of (FL)8hydrogels. The average breaking strain is 450±90% (n=16), Young’s modulus at 15% strain is 16±3 kPa (n=27), and breaking stress is 35±6 kPa (n=16). (b) Stressing–relaxation cycles from the same sample show that hydrogels built from (FL)8exhibit massive energy dissipation. It is of note that hydrogels show plastic deformation when stretched to higher strains due to the incomplete recovery of the hysteresis during consecutive stretching–relaxation cycles. (c). The hysteresis exhibited by (FL)8hydrogels can be largely recovered. (d) Kinetics of the hysteresis recovered shows a complex time course. The first∼60% hysteresis can be recovered within 2 s, while the remaining∼40% hysteresis is recovered much more slowly following an apparent double exponential kinetics. (e) Consecutive stress-strain curves of (FL)8hydrogels with different strains in 3 M GuHCl. Curves with different final strains are in different colours. Denatured (FL)8hydrogels show a much smaller Young’s modulus than native ones and do not exhibit appreciable hysteresis in stretching–relaxation cycles. Figure 5: Mechanical properties of (FL) 8 hydrogels. ( a ) Representative stress-strain curve of (FL) 8 hydrogels. The average breaking strain is 450±90% ( n =16), Young’s modulus at 15% strain is 16±3 kPa ( n =27), and breaking stress is 35±6 kPa ( n =16). ( b ) Stressing–relaxation cycles from the same sample show that hydrogels built from (FL) 8 exhibit massive energy dissipation. It is of note that hydrogels show plastic deformation when stretched to higher strains due to the incomplete recovery of the hysteresis during consecutive stretching–relaxation cycles. ( c ). The hysteresis exhibited by (FL) 8 hydrogels can be largely recovered. ( d ) Kinetics of the hysteresis recovered shows a complex time course. The first ∼ 60% hysteresis can be recovered within 2 s, while the remaining ∼ 40% hysteresis is recovered much more slowly following an apparent double exponential kinetics. ( e ) Consecutive stress-strain curves of (FL) 8 hydrogels with different strains in 3 M GuHCl. Curves with different final strains are in different colours. Denatured (FL) 8 hydrogels show a much smaller Young’s modulus than native ones and do not exhibit appreciable hysteresis in stretching–relaxation cycles. Full size image Furthermore, the majority of the hysteresis observed during tensile tests can be quickly recovered ( Fig. 5c ). Within 2 seconds, ∼ 60% of the observed hysteresis was recovered in the subsequent stretching cycle. The remaining 40% can be recovered following a complex and much slower time course ( Fig. 5d ). This suggests that the majority of domains that unfolded during stretching can refold efficiently, whereas a small fraction takes longer to refold. Such slow recovery for a small fraction of unfolded domains is responsible for the quasi-plastic deformation observed during consecutive stretching–relaxation cycles at higher strains ( Fig. 5b ). This also suggests that this quasi-plastic deformation is a time-dependent property. If the waiting time is long enough between consecutive cycles, FL hydrogels will not display noticeable plastic deformation. Previously, using GB1-resilin-based titin-mimetic artificial elastomeric proteins, we constructed protein hydrogels that exhibit mechanical properties that closely mimic the passive elastic properties of the muscles. GB1-resilin-based hydrogels usually fail at a strain less than 150% and only a very small number of GB1 domains unfold at higher strain, leading to energy dissipation [22] . Compared with such GB1-resilin-based hydrogels, FL hydrogels, we report here, are much more stretchy and tougher. We believe that forced unfolding of mechanically extremely labile FL domains and their subsequent hydrophobic collapse and aggregation in hydrogels are largely responsible for such excellent mechanical properties. To further confirm this conclusion, we carried out tensile tests on FL hydrogels in the presence of 3 M guanidine hydrochloride (GuHCl). CD measurements show that FL domains exposed to 3 M GuHCl are completely denatured (see Supplementary Fig. S3 ). When FL hydrogels are allowed to reach equilibrium in 3 M GuHCl solution, the hydrogels become transparent and swell significantly, suggesting that FL hydrogels have been converted into a cross-linked network of unfolded polypeptides ( Fig. 6 ). This also indicates that the aggregates formed by unfolded FL domains can disintegrate in high concentration of denaturants. 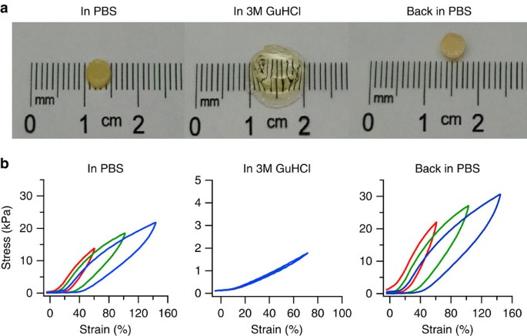Figure 6: Physical and mechanical properties of (FL)8hydrogels. Physical (a) and mechanical (b) properties of (FL)8 hydrogels reversibly tuned by GuHCL. In PBS, the hydrogel is opaque and shows a negative swelling ratio. Upon soaking in 3 M GuHCl, the hydrogel changes to transparent and swells significantly (with a swelling ratio 1780±200%). In addition, the hydrogel becomes highly compliant with a Young’s modulus of 1.7 kPa at 15% strain, and does not show appreciable hysteresis between stretching–relaxation curves. Upon removing GuHCl, the hydrogel reverts back to its original physical appearance, recovers its mechanical properties and becomes tough and highly stretchable. It is of note that the renatured hydrogels show increased Young’s modulus as compared with the original native hydrogels. Figure 6: Physical and mechanical properties of (FL) 8 hydrogels. Physical ( a ) and mechanical ( b ) properties of (FL)8 hydrogels reversibly tuned by GuHCL. In PBS, the hydrogel is opaque and shows a negative swelling ratio. Upon soaking in 3 M GuHCl, the hydrogel changes to transparent and swells significantly (with a swelling ratio 1780±200%). In addition, the hydrogel becomes highly compliant with a Young’s modulus of 1.7 kPa at 15% strain, and does not show appreciable hysteresis between stretching–relaxation curves. Upon removing GuHCl, the hydrogel reverts back to its original physical appearance, recovers its mechanical properties and becomes tough and highly stretchable. It is of note that the renatured hydrogels show increased Young’s modulus as compared with the original native hydrogels. Full size image Tensile tests ( Fig. 5e ) clearly show that such denatured hydrogels exhibit completely different mechanical properties: although they are still stretchable (with a typical breaking strain of ∼ 200%), they are much softer (with a Young’s modulus of 1.7±0.8 kPa at 15% strain, n =18) than native FL hydrogels and do not show appreciable energy dissipation. Such results are typical of networks constructed from random coil-like proteins [4] , and are consistent with the loss of folded three-dimensional structure of FL domains when exposed to the 3 M GuHCl solution. We also tested how the mechanical properties of the hydrogels will change when the denatured hydrogels are returned to conditions favourable for renaturation. It is of note that doing so restores the physical and mechanical properties of renatured hydrogels to a level that is very similar to the native hydrogels: this includes an opaque physical appearance, high stretchability and high toughness ( Fig. 6a,b ), strongly corroborating that these properties are indeed due to the forced unfolding and refolding behaviors of FL domains in FL hydrogels. Furthermore, it is significant that the Young’s modulus of the renatured hydrogels at 15% strain shows up to three times increase over the original gel ( Fig. 6b ). Although detailed mechanism is yet to be fully elucidated, it is likely that the formation of more aggregation of unfolded and collapsed FLs in close proximity is largely responsible for this increase in Young’s modulus of renatured FL hydrogels. During denaturation and renaturation cycles, it is reasonable to expect that some FL domains fail to refold after renaturation. Thus, renatured hydrogels contain more aggregated regions than original hydrogels, leading to increased Young’s modulus. Molecular origin of the unusual properties of FL hydrogels Based on these evidences, we propose the following mechanism detailing the origin of the unusual physical and mechanical properties exhibited by FL hydrogels ( Fig. 7 ). After photochemical cross-linking of the (FL) 8 polyprotein, the swelling force generated within the FL hydrogel in PBS is sufficient to trigger the unfolding of a significant fraction of mechanically labile FL domains in the FL hydrogels. Unfolding of FL domains leads to the increase in polymer length between the two adjacent cross-linking points and the relaxation of force experienced by individual (FL) 8 polyproteins. The unfolding of FL domains will cease until a new swelling equilibrium has been reached. PBS is a poor solvent for unfolded FL domains, as such unfolded FL domains will undergo hydrophobic collapse, which could lead to the aggregation of unfolded FL that are in close proximity and result in physical cross-linking. This effect leads to an intertwining chemically and physically cross-linked network structure. And such large aggregates formed by unfolded FL scatter light and give rise to the opaque appearance of native hydrogels. It is of note that the physical cross-linking proposed here is the result of the collapse and aggregation of forced unfolded FL domains, but not the intrinsic property of folded FL domains. Folded (FL) 8 does not form physically cross-linked network on its own. During stretching, both folded and unfolded FL domains are essential for the observed high stretchability and toughness of FL hydrogels. Upon stretching, force applied to the hydrogel will lead to the unfolding of more folded FL domains within the hydrogel. The massive length gain (27 nm per FL domain) and energy dissipation associated with FL unfolding lead to the high stretchability and toughness exhibited by the hydrogels. In addition, aggregates formed by unfolded FL domains can serve as force-bearing region in the hydrogel to increase the hydrogel’s mechanical strength and prevent microscopic crack propagation. Refolding of FL domains upon relaxation is responsible for the reversible hysteresis recovery demonstrated by the hydrogels. It is important to note that the number of FL domains in the FL polyprotein does not seem to affect the mechanical properties of FL hydrogels significantly, as hydrogels made of (FL) 4 , (FL) 12 and (FL) 16 show mechanical properties similar to those of (FL) 8 hydrogels ( Table 1 ). However, it remains unclear whether the size of the aggregates (or the number of unfolded/collapsed FL domains in a given aggregate) affects the mechanical properties of FL hydrogels. Future experiments will be needed to examine this important issue. 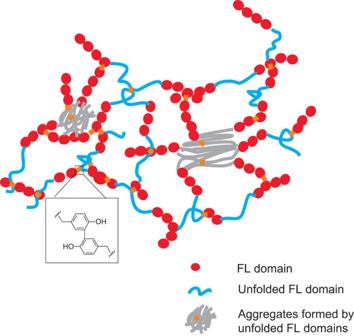Figure 7: Schematics of the structure of (FL)8-based hydrogels. The (FL)8-based hydrogels have intertwined chemically and physically cross-linked networks. Chemically cross-linked network is formed via a photochemical cross-linking strategy, which allows the cross-linking of two adjacent tyrosine residues into dityrosine adducts. Swelling force generated in the hydrogel results in the unfolding of a significant amount of FL domains, which then undergo hydrophobic collapse and form physically cross-linked large aggregates, giving rise to an opaque appearance of the hydrogel. Figure 7: Schematics of the structure of (FL) 8 -based hydrogels. The (FL) 8 -based hydrogels have intertwined chemically and physically cross-linked networks. Chemically cross-linked network is formed via a photochemical cross-linking strategy, which allows the cross-linking of two adjacent tyrosine residues into dityrosine adducts. Swelling force generated in the hydrogel results in the unfolding of a significant amount of FL domains, which then undergo hydrophobic collapse and form physically cross-linked large aggregates, giving rise to an opaque appearance of the hydrogel. Full size image Table 1 Mechanical properties of FL hydrogels. Full size table It has been recognized that incorporating easily ruptured structures, which act as sacrificial bonds, can significantly increase materials toughness. This mechanism is widely and effectively exploited in nature, mainly via force-induced unfolding of globular domains, to achieve desirable mechanical properties [11] , [12] , [13] , [14] , [15] , [41] , [42] . This idea has been used successfully to engineer novel tough and elastic synthetic polymer hydrogels [43] , [44] , [45] , however, surprisingly it has not been widely used in constructing protein-based hydrogels. Most synthetic proteinaceous hydrogels are constructed from unstructured or non-globular proteins [3] , [4] , [5] , [6] , [7] , [8] , [9] , [10] . Recently, using forced unfolding of titin-mimetic GB1-resilin-based elastomeric proteins as building blocks, we demonstrated the engineering of protein-based biomaterials that mimic the passive elastic properties of muscles [22] . Although energy dissipation in GB1-resilin biomaterials reflects many features observed for individual GB1 domains, the full potential promised by length increase and energy dissipation associated with unfolding of folded domains has not been realized [46] , as evidenced by the comparison between theoretic length increase of 900% upon unfolding of GB1 domains (ΔLc/L=18 nm/2 nm, where ΔLc is the length gain upon unfolding of GB1 and L is the original length in the folded state) versus ∼ 150% breaking strain for GB1-resilin biomaterials. Using forced unfolding of extremely mechanically labile globular domains as a design principle, here we have engineered a novel protein-based hydrogel that exhibits unusual physical and mechanical properties. Due to the low mechanical stability of FL domain, a significant fraction of FL domains in the hydrogel are unfolded by the force generated during swelling. Subsequent collapse and aggregation of unfolded FL lead to intertwining of physically and chemically cross-linked networks, entailing hydrogels with unusual physical and mechanical properties: a negative swelling ratio, high stretchability and toughness. These hydrogels are highly stretchable and tough, and show massive energy dissipation, which can be fully recovered upon relaxation via refolding of FL domains. These properties clearly demonstrate the potential of what forced unfolding of large amount of folded domains in hydrogels can offer for the engineering of protein-based biomaterials with desired mechanical properties at the molecular level. This work also clearly demonstrates that by carefully tuning the mechanical properties of folded domain, it is feasible to realize bottom-up, single-molecule level engineering of protein-based biomaterials. In this vein, we anticipate that an effective combination of de novo protein design, single-molecule mechanics and biomaterials construction will have a major impact on the engineering of unique biomaterials for potential applications in biomedical and tissue engineering. Protein engineering FL was de novo designed following published protocols [27] . The amino acid sequence of FL is: MGEFDIRFRT DDDEQFEKVL KEMNRRARKD AGTVTYTRDG NDFEIRITGI SEQNRKELAK EVERLAKEQN ITVTYTERGS LE. Its molecular weight is 9.69 kDa. FL domain is a redesigned variant of a previously published designer protein Di-I_5 (PDB code: 2KL8) and these two proteins share high sequence identity (75%). FL is predicted to assume the classical ferredoxin-like fold that is highly homologous to that of Di-I_5. Future endeavours are needed to obtain the crystal or NMR structure of FL. FL-M23C was designed based on the predicted structure of FL and was constructed using standard site-directed mutagenesis method. Polyprotein genes of (FL) 8 and (FL-M23C) 8 were constructed using standard molecular biology techniques following a well-established stepwise construction scheme [13] , [23] , which is based on the identity of the sticky ends generated by BamH I and Bgl II restriction enzymes. The polyprotein genes were subcloned into the expression vector pQE80L, and the resultant polyproteins carry an amino-terminal His-tag. The linker sequence between adjacent FL domains is -RS-, resulting from the restriction sites used in the constructing of the gene of (FL) 8 . The -RS- linker does not affect the thermodynamic properties of FL domain, as the thermodynamic properties of (FL) 8 are very similar to that of standalone FL domain (see Supplementary Fig. S3 ). For optical trapping experiments, we constructed a Cys-GB1-FL-Cys heterodimer. This heterodimer carries (His) 6 -Cys at the amino terminus and Lys-Cys at the carboxyl terminus, which facilitate protein purification using Co 2+ -affinity chromatography and the attachment of DNA handles at both termini for optical trapping experiments. Protein expression was carried out in Escherichia coli strain DH5α. Bacteria cultures were grown at 37 °C in 2.5% LB containing 100 mg/l ampicillin, and induced with 1 mM isopropyl-1-β- D -thiogalactoside when the optical density at 600 nm reached 0.8–1.0. Protein expression continued for 5 h at 37 °C. The cells were harvested by centrifugation at 6,000 r.p.m. for 10 min and cell lysis was done in PBS buffer containing protease inhibitor cocktail (0.3% v/v), lysozyme from egg white (1.25 mg ml −1 ), Triton X-100 (10 mg ml −1 ), DNaseI (5 μg ml −1 ) and RNase (5 μg ml −1 ). The supernatant containing soluble protein was isolated by centrifugation at 12,000 r.p.m., 4 °C for 1 h and purified by Co 2+ -affinity chromatography. The yield of (FL) 8 polyproteins was ∼ 80 mg l −1 of culture. The purity of the polyproteins was >90% as estimated from sodium dodecyl sulphate polyacrylamide gel electrophoresis (SDS–PAGE) analysed using AlphaEaseFC software (Version 4.0.0, Alpha Innotech Corporation, San Leandro, CA). Supplementary Fig. S2 shows the Coomassie blue G250 stained SDS–PAGE picture for the constructed polyprotein (FL) 8 . To prepare FL-based hydrogels, the purified polyproteins were dialyzed against deionized water for 16 h to completely remove the salt. The water was changed every 4 h during dialysis. Following dialysis, polyproteins were lyophilized. Single-molecule force spectroscopy measurements Single-molecule force spectroscopy measurements were performed using a custom built high resolution dual-trap optical tweezers setup with back-focal plane detection as described previously [47] . Sample preparation including the protein–DNA construct formation as well as the measurement procedure follow the same protocol as already reported [25] . Standard PBS was used as buffer at pH 7.4 (P4417, Sigma-Aldrich, St Louis, USA). Between different experiments trapping stiffnesses varied between 0.37 and 0.43 pN nm −1 . Data on the beads’ positions were recorded at a sampling rate of 20 kHz. After correcting the individual signals for cross-talk, final analysis was performed on the differential signal for a higher signal-to-noise ratio [48] . Force–extension relations of the protein–DNA construct were obtained from constant velocity pulling experiments. Fits to these data were done using the extensible worm-like chain model to describe the mechanics of the DNA handles in series with a worm-like chain model accounting for the elasticity contribution of the unfolded polypeptide chain allowing for the determination of the contour gain due to protein unfolding. Hidden–Markov analysis was used to separate the unfolded from the folded state within trajectories of constant pretension. Calculations of (force-dependant) transition rates and probabilities were conducted in accordance with the previous work [25] . Hydrogel preparation Hydrogels made of (FL) 8 , (FL-M23C) 8 or (FL-C) 8 were prepared following protocols described previously [22] . A typical cross-linking reaction mixture contained 200 mg ml −1 of polyprotein, 200 μM [Ru(bpy) 3 ] 2+ Cl 2 and 50 mM ammonium persulfate in PBS buffer. Trapped air bubbles were removed by centrifugation at 12,000 r.p.m. for 3 min. The solution was cast into a custom-made plexiglass mould with an inner diameter of 8 mm, outer diameter of 10 mm and height of 3 mm. The sample was then irradiated for 10 min using a 200 W fibre optical white light source at room temperature placed 10 cm away from the mould. The ring-shaped biomaterial was then taken out from the mould and stored in 10 mM PBS buffer containing 0.05% (w/v) sodium azide to prevent microbial growth. These chemically cross-linked hydrogels are opaque and show superior long-term stability, with no noticeable erosion observed in sodium-azide-containing PBS buffer over a period of one year. The degree of tyrosine cross-linking in the hydrogels was estimated following a previously established method based on dityrosine fluorescence [49] . We found that ∼ 13% tyrosine residues in FL domains are cross-linked into dityrosine adducts (including intra- and intermolecular cross-linking) in the hydrogels. Circular dichroism measurements CD spectra were recorded on a Jasco-J810 spectropolarimeter flushed with nitrogen gas. The spectra were recorded in a 0.1 cm path length cuvette at a scan rate of 100 nm per min. For each protein sample, an average of three scans was reported. Protein samples were measured in 0.5 × PBS at pH 7.4, where data were corrected for buffer contributions. The chemical denaturation curves were measured by monitoring the ellipticity of FL at 220 nm at 25 °C as a function of chemical denaturant concentration (GuHCl). To obtain thermodynamics stability of FL ( ), the chemical denaturation curves were fitted by nonlinear square fits using a two-state unfolding and linear extrapolation model [50] . Swelling measurement and tensile test For swelling measurements, ring-shaped hydrogels were weighted immediately after being taken out of mould, and the weight was recorded as W 0 . Hydrogels were then soaked in PBS at the room temperature. After certain time, the hydrogel rings were taken out of PBS buffer, blotted onto tissue paper to remove excess buffer and weighted as W t . The swelling ratio was calculated according to the formula: Swelling ratio (%)=[( W t − W 0 )/ W 0 ] × 100%. Tensile tests were performed using an Instron-5965 tensometer with a 5-N load cell and a custom-made force gauge. The ring-shaped biomaterial was stretched at an extension rate of 25 mm min −1 in PBS in most tensile tests, with the exception of hysteresis recovery experiments, where a pulling rate of 200 mm min −1 was used. For technical considerations, ring-shaped biomaterial specimens were used [40] . The local slope at 15% strain on the extension curve was taken as the modulus at 15% strain reported in the study. In order to compare our results with those reported in the literature, our tensile testing were carried out at 22 °C. It is of note that in order to evaluate the potential use of FL hydrogels for in vivo applications, tensile testing carried out at 37 °C will be required. For tensile testing of break point, no special preconditioning was conducted. Most hydrogel samples were loaded directly to failure. A small fraction of hydrogel samples were subjected to tensile testing first, then equilibrated in PBS buffer overnight before they were loaded to failure. In both cases, we did not observe obvious difference. SEM measurements For SEM imaging experiments, FL hydrogels were shock-frozen in liquid nitrogen immediately after being taken out of mould. Such samples were designated as hydrogels without deswelling. For hydrogels after deswelling: hydrogels were put in PBS after being taken out of mould and equilibrated for 30 min. After the hydrogel samples were taken out of PBS and blotted onto tissue paper to remove excess buffer, hydrogels were shock-frozen in liquid nitrogen. Frozen samples were quickly transferred to a freeze dryer and lyophilized for 12 h. The dry samples were then carefully fractured in liquid nitrogen and fixed on aluminium stubs. The surface of the samples was coated with 5 nm gold before SEM observation. SEM imaging of the FL hydrogels was performed using a Hitachi S4700 scanning electron microscope. Cysteine shotgun fluorescence labelling by IAEDANS Procedures for Cysteine shotgun fluorescence labelling experiments by IAEDANS were adapted from those described previously [38] . Cysteine shotgun fluorescence labelling for (FL) 8 , (FL-M23C) 8 and (FL-C) 8 was done at a protein concentration of 125 μM, where a 10-fold excess of IAEDANS was used. The labelling reaction proceeded in the dark at 20 °C for 2 h either in PBS with 5 mM Tris-(2-carboxyethyl)phosphine (TCEP) (for folded proteins) or 7 M GuHCl with 5 mM TCEP (pH 7.4) (for denatured proteins). The labelled protein was then purified by Co 2+ -affinity chromatography. Eluted proteins were analysed using SDS–PAGE. To check whether more FL-M23C were unfolded during stretching, we carried out Cysteine shotgun fluorescence labelling of hydrogels under different strains. The labelling reaction was carried out in dark at room temperature for 2 h in PBS buffer containing 5 mM TCEP and 2 mM IAEDANS in a custom-made device where the hydrogel was held at a specific strain. As a control experiment, a (FL-M23C) 8 -based hydrogel soaked in 7 M GuHCl (containing 5 mM TCEP, pH 7.4) was also fluorescently labelled using IAEDANS. After labelling, the hydrogels were transferred to PBS buffer containing 5 mM β-mercaptoethanol (to quench the labelling reaction) and gently shaken at 30 r.p.m. on an orbital shaker for 5 h. During this time, the PBS buffer (containing 5 mM β-mercaptoethanol) was changed five times. The dye-labelled hydrogels were stored in PBS buffer at 4 °C before tryptic digestion. Fluorescence measurements of the labelled hydrogels To quantify the fluorescence intensity of labelled hydrogels by IAEDANS, we first carried out tryptic digestion of hydrogels at 37 °C for 5 h in a buffer containing 25 mM NH 4 HCO 3 , 10 mM CaCl 2 , 1 M Guanidine-HCl and 10 mM dithiothreitol. Trypsin, which amounts to 5% of the hydrogel’s weight, was used in the digestion reaction. The unlabelled (FL-M23C) 8 hydrogel was digested in the same way as a control. After trypsin digestion, 100 μl of the digested reaction mixture was diluted to 1 ml using PBS buffer, and its fluorescence emission spectrum was then recorded using a Varian Eclipse fluorescence spectrometer using an excitation wavelength of 336 nm. The fluorescence intensity of IAEDANS at 490 nm was used as a semi-quantitative measure of the concentration of IAEDANS-modified cysteine residues in hydrogels. Liquid chromatography tandem mass spectrometry The tryptic peptide mixture containing approximately 10 μg of peptide was desalted on homemade C18 stop-and-go-extraction tips (StageTips) [51] . The eluent was then dried and reconstituted in 6 μl of 0.5% acetic acid. Separation and identification of peptides were performed on an Agilent 1100 nano-HPLC system (Agilent, Santa Clara, CA) using a 15 cm long, 75 μm inner diameter fused silica column packed with C18 reverse phase beads (3 μm particle size). The HPLC system was coupled to an FT-ICR tandem mass spectrometer (LTQ-FT, Thermo Electron Corporation, Waltham, MA) running in positive charge mode. Water and acetonitrile with 0.5% acetic acid were used as a mobile phase to perform gradient elution. Raw spectra were searched for IAEDANS-modified peptides using MaxQuant 1.3.0.5 integrated with Andromeda peptide search engine [52] . Search parameters were set as follows: variable modifications: IAEDANS (customized, C 14 H 14 N 4 O 2 S, mass=306.0674); multiplicity: 1; enzyme: trypsin/P; first search p.p.m: 20; main search p.p.m: 6; max missed cleavage: 3; MS/MS tolerance: 0.5 Dalton; FASTA file was created to only contain the M23C sequence; peptide FDR: 0.1. Fragment ions were identified automatically by MaxQuant and verified manually. Additional matching fragments ions were identified through manual assignment. How to cite this article: Fang, J. et al . Forced protein unfolding leads to highly elastic and tough protein hydrogels. Nat. Commun. 4:2974 doi: 10.1038/ncomms3974 (2013).